Deep resequencing reveals excess rare recent variants consistent with explosive population growth Accurately determining the distribution of rare variants is an important goal of human genetics, but resequencing of a sample large enough for this purpose has been unfeasible until now. Here, we applied Sanger sequencing of genomic PCR amplicons to resequence the diabetes-associated genes KCNJ11 and HHEX in 13,715 people (10,422 European Americans and 3,293 African Americans) and validated amplicons potentially harbouring rare variants using 454 pyrosequencing. We observed far more variation (expected variant-site count ∼ 578) than would have been predicted on the basis of earlier surveys, which could only capture the distribution of common variants. By comparison with earlier estimates based on common variants, our model shows a clear genetic signal of accelerating population growth, suggesting that humanity harbours a myriad of rare, deleterious variants, and that disease risk and the burden of disease in contemporary populations may be heavily influenced by the distribution of rare variants. Models of human genetic diversity have an important role in both population genetics and genetic epidemiology, and considerable effort has been expended to characterize human genetic diversity by directly sequencing DNA from large population samples (for example, refs 1 , 2 , 3 , 4 ) and from the ongoing 1000 Genomes and Personal Genomes projects [5] , [6] . To study the distribution and role of truly rare variants, it is necessary to sequence extremely large numbers of individuals, a project that has only recently become feasible. An inherent problem with such a deep resequencing effort is distinguishing actual rare genetic variants from stochastic sequencing errors, which will occur at almost every site if enough individuals are resequenced. Regenotyping the sites of potential rare variants can mitigate this uncertainty; however, for large-scale studies, there are so many rare single-nucleotide polymorphism (SNP) calls that regenotyping all of them becomes cost prohibitive. Another approach is to focus on variants for which the sequence evidence is very strong. This worked well for Sanger sequencing in the HapMap project [7] ; however, crucially, the HapMap project had a much smaller sample size and targeted high-confidence calls of common SNPs for inclusion on a SNP chip. False-negative SNP calls were a minor concern for HapMap, whereas for a comprehensive catalogue of rare variation, it is important to minimize them. Therefore, to catalogue rare variants in a thorough and cost-effective manner, in this study we assign probabilities to genotype calls, explicitly estimating our uncertainty for each call. This approach differs from earlier methods [8] , [9] by using the overlapping genotypes of the (Sanger) ENCODE and (SNP Chip) HapMap projects to train a Dirichlet mixture which relates genotypes to the distribution of phred probability scores. As we assign probabilities to all genotype calls, all analyses of the genotypes are also probabilistic, carrying the genotype uncertainty forward to quantitative estimates of the resulting uncertainty in our sitefrequency spectrum (SFS) and population-genetic estimates. In this study, we selected genes KCNJ1 1 and HHEX for resequencing in 13,715 individuals. Such a large sample made some unique population-genetic calculations possible, such as a model of the growth rate of the European population over the last few thousand years. Earlier population-genetic models of European population growth [10] based their estimates on higher-frequency variants than the bulk of variants ascertained in our study. By estimating the distribution of times at which a variant of a given contemporary frequency might have plausibly arisen in the ancestral population, we have been able to compare our growth-rate estimate with earlier estimates. We were also able to separately estimate mutation rate and demographic parameters, which are normally confounded in equilibrium population genetics [11] , and estimate the mutation rate specific to each gene locus, using a population-genetic model similar to those described in Wakeley and Takahashi [11] and Boyko et al . [12] Our SFS showed far more rare variation than would have been predicted by classical models of population genetics, and our population genetics calculations established a clear genetic signal of a recent acceleration in European population growth. Sequencing assay We resequenced these genes in 13,715 ARIC (Atherosclerosis Risk In Communities) individuals (3,293 African Americans and 10,422 individuals of European ancestry, Supplementary Methods ). We applied Sanger sequencing of PCR products from genomic DNA from 50 amplicons covering the coding regions, introns and near flanking regions (see Supplementary Methods ). We achieved excellent sequence coverage of the loci, and called variant sites in a way that assigned probability scores to each (see Methods). To quantify the rate of sequencing error, we validated potential rare variants by barcoding and pooling of the relevant PCR amplicons, and then submitted them en masse to 454 Roche sequencing. We validated 216 sites, the majority of which were high-probability variant calls in our initial genotyping. We used the results of this exercise to calibrate our genotype probabilities with their accuracy in calling rare variants ( Supplementary Methods ). There are many variants with predicted biological impact: combined over the two genes, there are 35 sites with a probability of at least 0.35 that the genotype varies in a way that would change the protein product; 19 of these are identified by PolyPhen [13] as potentially damaging, on the basis of cross-species sequence conservation at those sites. 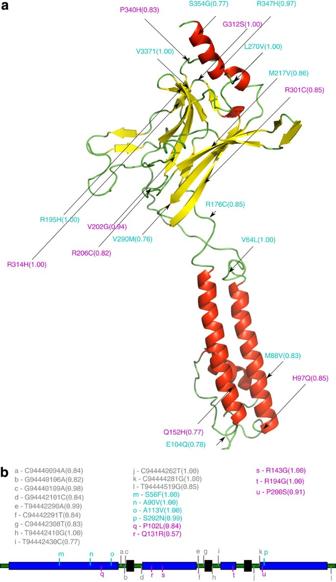Figure 1: Physical location of selected variants. For each variant shown, the figure shows the reference residue, the location, the variant residue and, in parentheses, the variant's posterior probability. Variants identified by Polyphen13as potentially damaging to the protein product are shown in magenta, others are in cyan. (a) Variants that change the protein structure inKCNJ11. (b) Variants inHHEX. No sufficiently homologous crystal structure forHHEXis available for homology modelling; hence, we show the gene structure instead. Blue regions depict exons. Green regions depict neighbouring intronic/untranslated regions (30 base pairs in both directions). Black bars indicate excluded intronic sequence. Non-coding variants are shown in grey, and show the reference allele, the build 36 coordinate on chromosome 10, the variant allele and the posterior probability of the variant. Figure 1 is a survey of the potentially damaging variants, and gives the probabilities that the variants are present at the indicated sites. By contrast, dbSNP [14] ( http://www.ncbi.nlm.nih.gov/projects/SNP/ ) reports just two and ten missense SNPs in HHEX and KCNJ11 , respectively. Although a PolyPhen call of 'damaging' is not definitive, this observation of rare variation at a large number of evolutionarily conserved sites is consistent with the expectation that rare, recent variants are more randomly distributed than common variants, because selection pressures have had less time to act on them. The KCNJ11 protein structure in Figure 1 was determined by homology modelling using SWISS-MODEL [15] , and covers residues 33–357 (out of a total of 390 residues). There were other protein-changing KCNJ1 variants at sites not covered by the model. Those identified by Polyphen as benign were V13M, R29H and L361F (posterior probabilities 1.00, 0.35 and 0.85, respectively). Those identified as potentially damaging were E23K, R31W, R371H, P374R and S385C (posterior probabilities 1.00, 0.36, 0.97, 0.96 and 1.00, respectively). No sufficiently homologous crystal structure for HHEX is available for homology modelling; therefore, we show the gene structure instead ( Fig. 1b ). Figure 1: Physical location of selected variants. For each variant shown, the figure shows the reference residue, the location, the variant residue and, in parentheses, the variant's posterior probability. Variants identified by Polyphen [13] as potentially damaging to the protein product are shown in magenta, others are in cyan. ( a ) Variants that change the protein structure in KCNJ11 . ( b ) Variants in HHEX . No sufficiently homologous crystal structure for HHEX is available for homology modelling; hence, we show the gene structure instead. Blue regions depict exons. Green regions depict neighbouring intronic/untranslated regions (30 base pairs in both directions). Black bars indicate excluded intronic sequence. Non-coding variants are shown in grey, and show the reference allele, the build 36 coordinate on chromosome 10, the variant allele and the posterior probability of the variant. Full size image Variant counts The data reveal a vast number of rare variants. By drawing repeated samples from the genotype probabilities, counting the number of variants in each such sample and taking the average of these counts, we compute the expected number of variant sites in this sample to be 578.6 (s.d.=7.6), with 316.9 in HHEX and 261.7 in KCNJ11 (see descriptions of loci and count sampling in Methods). In sub-samples, the number of singleton-variant sites observed increases almost linearly with sample size ( Fig. 2 , which shows the counts for variants found in the European-American cohort). 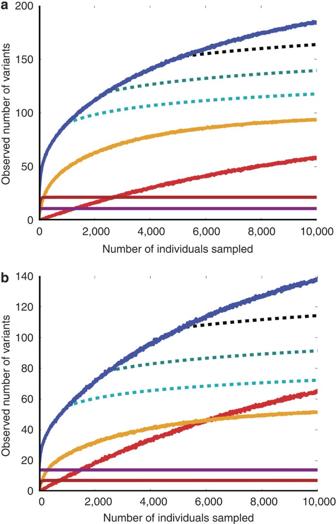Figure 2: Number of variants as a function of sample size. Counts of the number of observed segregating sites as a function of sample size for (a)HHEXand (b)KCNJ11. Solid blue line shows the total number of segregating sites. Red shows singletons, and yellow, brown and purple lines show the numbers of variants with relative minor allele frequency <0.01, 0.01–0.05 and more than 0.05, respectively. Roughness in these curves indicates stochasticity in the number of variants observed across multiple sample populations. Dashed lines show extrapolations of the expected number of segregating sites in larger samples according to Watterson's classical estimate. In all cases, we found far more segregating sites at larger sample sizes than Watterson's estimate would have predicted. Figure 2: Number of variants as a function of sample size. Counts of the number of observed segregating sites as a function of sample size for ( a ) HHEX and ( b ) KCNJ11 . Solid blue line shows the total number of segregating sites. Red shows singletons, and yellow, brown and purple lines show the numbers of variants with relative minor allele frequency <0.01, 0.01–0.05 and more than 0.05, respectively. Roughness in these curves indicates stochasticity in the number of variants observed across multiple sample populations. Dashed lines show extrapolations of the expected number of segregating sites in larger samples according to Watterson's classical estimate. In all cases, we found far more segregating sites at larger sample sizes than Watterson's estimate would have predicted. Full size image The full spectra for both population groups are shown in Supplementary Figure S1 . Spectra for synonymous and non-synonymous variants are shown in Supplementary Figure S2 . 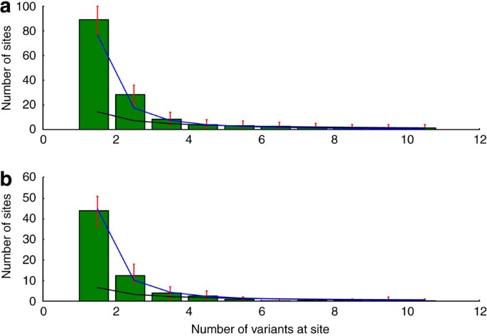Figure 3: Site-frequency spectra. Site-frequency spectra in (a)HHEXand (b)KCNJ11over 'neutral sites' (see Methods) in the two genes for the European sub-population. Thexaxis depicts the number of variants observed at a site; theyaxis depicts the expected number of sites at which that many variants were seen. Green bars show the expected number of sites, as determined by sampling from the posterior genotypic distributions for each sampled individual, and error bars show the 99% confidence intervals from these samples. The black line shows the expected SFS spectrum, given the Wright–Fisher constant population size model and mutation rate Θ estimated by Watterson's method (Equation 4.16, Hartl & Clark (2007)) The blue line shows the mean posterior SFS given the population model used to calculate the mutation rate inFigure 4. The spectra for non-coding regions seem to be very similar to those in Figure 3 , because non-coding sites dominate the class of sites in which nucleotide variation can have no impact on the protein residue sequence. Figure 3: Site-frequency spectra. Site-frequency spectra in ( a ) HHEX and ( b ) KCNJ11 over 'neutral sites' (see Methods) in the two genes for the European sub-population. The x axis depicts the number of variants observed at a site; the y axis depicts the expected number of sites at which that many variants were seen. Green bars show the expected number of sites, as determined by sampling from the posterior genotypic distributions for each sampled individual, and error bars show the 99% confidence intervals from these samples. 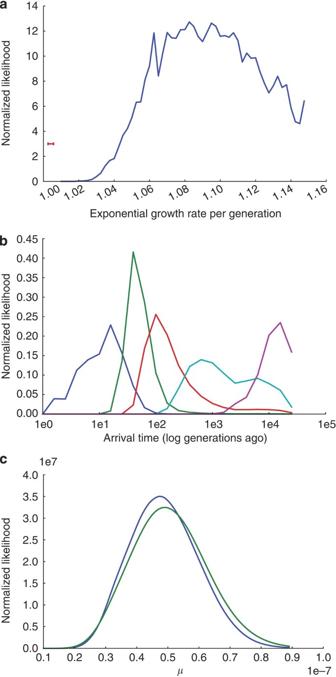Figure 4: Mutation rate estimates. These estimates are based on drawing an average over 100 coalescent trees per grid point. (a) Estimated marginal posterior distribution over growth rates per generation during the exponential growth phase. Red error bar in the lower left-hand corner shows the 95% confidence interval of the growth rate in the European lineage estimated in Table 1 of Gutenkunstet al.10which is much lower, because the more common variants used in that estimate pertain to a more remote time in our history. (b) Estimated marginal posterior distributions on the time when variants of various relative minor allele frequencies arose in the population, relative to the logarithm of number of generations ago. Blue, green, red, cyan and magenta lines correspond to distributions for variants with relative minor allele frequency (RMAF) of 5×10−5, 5×10−4, 5×10−3, 5×10−2and 5×10−1, respectively. A RMAF of 5×10−5corresponds to singletons in our data set, which, according to our model, mostly arose in the last 2,500 years. Most previous analyses have dealt with SNPs with a RMAF on the order of 5×10−2, corresponding to much earlier mutations. (c) Estimated marginal posterior distribution over mutation rates given the SFS in the two genes. Blue and green lines are forHHEXandKCNJ11, respectively. The black line shows the expected SFS spectrum, given the Wright–Fisher constant population size model and mutation rate Θ estimated by Watterson's method (Equation 4.16, Hartl & Clark (2007)) The blue line shows the mean posterior SFS given the population model used to calculate the mutation rate in Figure 4 . Full size image Population genetic calculations We fit a model of exponential growth to the SFS (see Fig. 3 ) of our European-American sample (see Methods). To avoid complications from evolutionary selection pressures, such as those described in Ohta [16] , we restricted this analysis to sites at which no selection pressure is to be expected (Methods). The excess of rare variants in HHEX and KCNJ11 fits well with this model ( Fig. 3 ), giving a mean posterior growth rate of 1.094 (that is, an increase of 9.4%) per generation ( Fig. 4a ). Figure 4: Mutation rate estimates. These estimates are based on drawing an average over 100 coalescent trees per grid point. ( a ) Estimated marginal posterior distribution over growth rates per generation during the exponential growth phase. Red error bar in the lower left-hand corner shows the 95% confidence interval of the growth rate in the European lineage estimated in Table 1 of Gutenkunst et al . [10] which is much lower, because the more common variants used in that estimate pertain to a more remote time in our history. ( b ) Estimated marginal posterior distributions on the time when variants of various relative minor allele frequencies arose in the population, relative to the logarithm of number of generations ago. Blue, green, red, cyan and magenta lines correspond to distributions for variants with relative minor allele frequency (RMAF) of 5×10 −5 , 5×10 −4 , 5×10 −3 , 5×10 −2 and 5×10 −1 , respectively. A RMAF of 5×10 −5 corresponds to singletons in our data set, which, according to our model, mostly arose in the last 2,500 years. Most previous analyses have dealt with SNPs with a RMAF on the order of 5×10 −2 , corresponding to much earlier mutations. ( c ) Estimated marginal posterior distribution over mutation rates given the SFS in the two genes. Blue and green lines are for HHEX and KCNJ11 , respectively. Full size image The variance in this estimate is high; however, combined with earlier demographic estimates, our growth-rate estimate gives a clear genetic signal that over the last few millennia, the rate of population expansion has accelerated substantially. Because previous genomic studies of human population samples have been based on either resequencing a small group of individuals or on HapMap SNPs ascertained with a bias towards common variation, these have only captured the distribution of common variants (relative minor allele frequency ∼ 0.05). As shown in Figure 4b , we find that most of the variants in this part of the frequency spectrum arose about 100–3,000 generations ago, or about 2,500–75,000 years ago, assuming 25 years per generation. In the exceptionally large sample resequenced here, singletons correspond to mutations that arose during the last ∼ 100 generations ( Fig. 4b ), and thus carry information about the demographics of Europe after its widespread adoption of agriculture [17] . Despite relying on shallower regenotyping data, earlier studies [10] also found a good fit to an exponential growth model, but with the substantially lower modal growth rate of 1.004 per generation. Our posterior distribution implies that the growth rate is bound below by 1.015; hence, by comparing our results with those of Gutenkunst et al . [10] , we conclude that Europe's population growth rate accelerated substantially over the last 2,000 years, and our mean posterior growth-rate estimate implies an acceleration by more than an order of magnitude. Reliable census estimates of Europe's population begin around 1550 [18] , and the growth rate in Europe since 1600 has been ∼ 11.5% per generation (estimated from Table 1.3 of Livi-Bacci [19] , assuming 25 years per generation). This suggests that in future, even deeper resequencing efforts will reveal an SFS with even greater proportions of rare and missense variants with potential consequences for human health. Mutation rate estimates Our model yields mean mutation rate estimates of ∼ 4.9×10 −8 and ∼ 5.1×10 −8 mutations per site per generation for HHEX and KCNJ11 , respectively ( Fig. 4c ). These estimates are in approximate agreement with earlier genome-wide estimates based on human–chimpanzee divergence [20] or de novo mutations in monogenic disorders [21] ; however, our extremely deep sampling has enabled estimates local to each gene. These estimates will become more precise in the future using samples across larger sets of genes (which will make the demographic parameter estimates more precise) and larger groups of people (which will make all parameter estimates more precise). The majority of the variants we found are extremely rare and could only have been captured by the kind of exceptionally deep resequencing described here ( Figs 1 and 2 ). From the perspective of classical population genetics for stable populations, this abundance of rare variation is surprising: the expected number of singletons in our data is at least five times greater than the standard Wright–Fisher model [22] would predict, and we find a nearly linear increase in the number of singletons as the sample size grows, whereas the classic theory for stable populations predicts that discovery of new variant sites will rapidly saturate as the sample size increases. This departure from the expected distribution suggests recent explosive human population growth, which has produced gene genealogies with a preponderance of short, recent genealogical branches. Assuming mutations are uniformly distributed over these genealogies, most mutations will have fallen on those very recent branches; thus, most variants will appear in only a few contemporary individuals. We thus predict that rare human genetic variation will tend to be more damaging than the common variants that have been the main focus of genetic studies up to this point. This is because in a sufficiently large sample, every human gene is likely to harbour many rare variants that have arisen so recently that selection can have influenced the frequencies of only the most severely deleterious alleles ( Fig. 1 ). We also predict that all individuals carry multiple loss-of-function alleles in their genome [21] , [23] , [24] , [25] , [26] . Although these predictions must be tested in a future assay, a simple calculation assuming a conservative mutation rate of 1×10 −9 still implies that the human genome of ∼ 3×10 9 sites is saturated with mutations arising just in the current human generation of 6.7×10 9 people. This supports the concerns raised by Lynch [21] regarding burgeoning human “mutational load” and bears on the 'missing heritability' still unexplained by genome-wide association studies [27] . This myriad of rare but potentially large-effect variants are embedded in diverse gene regulatory pathways, suggesting that considerable phenotypic differences may arise from low-frequency genetic architectures [28] , [29] . Knowledge of these variants may provide good individual phenotypic predictive ability within families, but their individual rarity in a population will mean that they will have very low population-attributable risk. This suggests that the best scale for inference about the genetics of complex disorders may be individuals with genomic regions of highly shared ancestry, including the family unit itself. DNA sequencing Using traditional Sanger fluorescent dideoxy methods on ABI 3730 capillary sequencers, we resequenced HHEX and KCNJ11 in the ARIC cohort. Primers were designed to yield tiled amplicons across the full HHEX (7.9 kb) and KCNJ11 (5.5 kb) genes, including exons and introns and 1.2 kb upstream of the transcriptional start site, so that the coverage began for HHEX at global coordinate (build 36) 94438570 and ended at 94446433, and for KCNJ11 began at 17362320 and ended at 17367885. See Supplementary Table S1 for primer sequences. The design was successful in providing coverage for more than 90% of each gene. Low-quality sequence reads and amplicons that failed to map to the related amplicon in the human reference sequence were removed, leaving 50 amplicons in overlapping tiles across the genes. There was one region that failed to map in HHEX that spanned 442 bp, including 100 bp of the coding region. There were three such regions in KCNJ11 : one spanning 43 bp, another spanning 59 bp and a third spanning 537 bp, none of which were in the coding regions. These mapping failures were likely caused by very high GC content interspersed with simple tandem repeats. Trace files have been deposited in the NCBI trace archive under center_name="bcm" and center_project="rhicf". Genotype calling Rare variants are a challenge to score by Sanger sequencing, because they are likely to be present in a population sample only as heterozygotes. Heterozygotes are difficult to distinguish from aberrations in Sanger sequencing data, because the PCR products in the sequencing gel come from both chromosomes; hence, heterozygous genotypes appear as a superposition of the two alleles. In particular, a heterozygous SNP resembles a 'double peak' in the Sanger trace file, but so do certain types of noise. The most popular program for analysing Sanger sequence data, phred [30] , was designed for haploid organisms, and explicitly treats such superposition as a sign of noisy data; hence, it cannot be used to directly identify heterozygous SNPs. Various approaches have been used to overcome this limitation by using only phred to highlight the double peaks, then analysing them separately. However, phred was carefully trained on a substantial corpus of sequencing data, although from haploid clones; therefore, we developed a way to make use of that previous training to evaluate each of the peaks by masking one allele to render our diploid sequence haploid-like (detailed below). In our approach, we effectively separated the colour channels at double peaks to obtain separate phred calls for each possible nucleotide in such a way that, as much as possible, phred would interpret them as clean haploid peaks. The distribution of phred software comes with the source code; hence, we were able to modify the way it responds to double peaks in the trace files: we programmed it to zero out each peak channel so that the other peak could be rescored using phred's standard machinery without being confounded by the superposition. Phil Green and Brent Ewing have very generously agreed to permit the use and distribution of our patch to phred, and to continue providing the version of the source code to which it applies (version 0.020425.c.) Once modified, phred reports up to three scores for each of the peaks in a trace file: it always reports the standard phred score, and in the case of a double peak it potentially also reports the two scores obtained by zeroing out each of the peak channels. There is only one instance when these two extra scores are censored: it often happens that the dominant channel for one peak 'runs on' into an overlap with the next peak, creating a double peak that has nothing to do with genetic variation. We programmed phred to ignore a double peak if it immediately follows a peak on the same channel as its minor peak, and the amplitude of the minor peak is <20% of that of the major peak. A number of individuals genotyped in the HapMap 3 project were also sequenced in the ENCODE project [31] , and we used this comparison data to train the priors in our model. We took the HapMap 3 genotypes as the gold standard, and at 830 sites with both HapMap 3 genotypes and Sanger sequence data we ran our modified phred. For each site with a given genotype g, as reported by HapMap 3, we counted how many times each type of peak was observed in the ENCODE trace files at that site. Trace files from the reverse strand were associated with the complementary genotype. This gave us a set of per-site counts for types of peaks. We used these counts to train Dirichlet mixture priors T g (on the types of peaks observed at a site with given genotype g) and S gp (on the phred scores observed at a site with genotype g and peak type p) in much the same way as described in Sjölander et al . [32] , except that we considered priors with up to six mixture components and, for each number of mixture components, we sampled mixture weights and pseudocounts using Hamiltonian Markov Chain Monte Carlo [33] , using a flat hyperprior on the mixture weights and exponential distributions of mean 1 on the pseudocounts for each component. From among the six priors constructed this way (one for each possible number of mixture components), we chose the one with the highest total probability (that is, the probability of the data given the constructed prior multiplied by the probability of the prior given the hyperprior) and used that as T g. Similarly, for each genotype g and peak type p, we constructed counts for the scores associated with them as follows: for every site where this genotype and peak type was observed, we counted the number of times each phred score was observed in people with that genotype and peak type at that site. We trained a mixture prior S gp from these counts in the same way as we trained T g. We used this prior in a Markov Chain Monte Carlo series at each site that also accounted for the population-level genotype frequencies at the site, so that it takes stronger evidence to call rarer genotypes. The software application, SnppnS, is available as Supplementary Software or can be downloaded from http://micortex.org/software.php . Sampling of site-frequency spectra Because we generate genotype probability distributions rather than categorical genotype calls, there is some uncertainty in the SFS for our genetic data. To generate Figure 3 , we drew samples from the posterior genotype distributions for every position, and used these categorical genotypes to generate an SFS. We repeated this sampling 1,000 times. The error bars in Figure 3 represent the 99% confidence intervals on the site counts for each bin. To show concordance with the predicted SFS from the population genetics calculation in the next section, the spectra in Figure 3 show the frequency distribution only for variants at the same set of 'neutral' sites used in that calculation: wobble sites or those at least 30 base pairs from a coding region. So that each site would come from a population of the same size, in the European (African)-American sample, we ignored all sites called in fewer than 10,000 (3,000) people. For sites called in more than 10,000 (3,000) people, we randomly sampled a group of 10,000 (3,000) and drew our counts from that. Population genetics calculations To minimize the complications of admixture, we restricted this analysis to the European-American sample. Our model thus has three parameters that we needed to search over: the mutation rate μ , the estimated population size at the start of ARIC, N , and the growth rate during the exponential phase r . We did a grid search over these parameters using the following values: μ : 10 −8 per site per generation, up to 9×10 −8 , in steps of 10 −9 ; r : 1.01 per generation, up to 1.15 per generation in steps of 0.0025; and N : 2×10 5 , up to 4×10 6 , in steps of 10 5 . Because we were comparing with the growth-rate estimate in Gutenkunst et al ., [10] of 1.004 per generation, we also separately computed the following likelihoods for r in the vicinity of that, and found them to be negligible. We fit these parameters to the SFS from our genetic data. To avoid confounding by selection pressures, for this calculation we used an SFS restricted to either sites that were at least 30 base pairs from an exon or third-position sites in codons that could mutate to any nucleotide with no impact on the protein product. We also ignored all sites with genotype calls for fewer than 10,000 people. For sites called in more than 10,000 people, we computed their contributions to the SFS from random samples of 10,000 individuals. We were thus able to assume for this calculation that we had full sample data in exactly 10,000 people at all sites considered. Our calculation is similar to those described in Wakeley and Takahashi [11] and Boyko et al ., [12] and is described in the Supplementary Methods . How to cite this article: Coventry, A. et al . Deep resequencing reveals excess rare recent variants consistent with explosive population growth. Nat. Commun. 1:131 doi: 10.1038/ncomms1130 (2010).